Light focusing in the Anderson regime Anderson localization is a regime in which diffusion is inhibited and waves (also electromagnetic waves) get localized. Here we exploit adaptive optics to achieve focusing in disordered optical fibres in the Anderson regime. By wavefront shaping and optimization, we observe the generation of a propagation-invariant beam, where light is trapped transversally by disorder, and show that Anderson localizations can be also excited by extended speckled beams. We demonstrate that disordered fibres allow a more efficient focusing action with respect to standard fibres in a way independent of their length, because of the propagation-invariant features and cooperative action of transverse localizations. Adaptive techniques have turned around optics allowing not only to correct aberrations in the image formation but also to focus light beams through curtains of dielectric scatterers [1] , [2] , [3] by employing the most transmitting modes [4] . The focusing may be achieved by wavefront shaping, using spatial light modulators (SLMs) and applying a specific phase distribution to the input beam to correct the random delay imposed by the diffusive propagation. Focusing by wavefront shaping has opened the way to many novel applications [5] , [6] , [7] as it can be realized in any disordered structure, even if, so far, it has been studied only within the diffusive regime, in the absence of mechanisms of wave localization. It is well accepted that if the strength of disorder increases beyond a critical value, a transition called Anderson localization [8] , [9] , [10] takes place. In the proximity of this regime, there is a drastic reduction of diffusion, and ultimately an absence of transport. Being originated by interference, Anderson localization is common to all kind of waves and has been demonstrated for matter waves [11] , sound [12] and entangled photons [13] . For light, it is difficult to achieve localization in three dimensions (3D) [14] because the scattering strength has to be strong enough to satisfy the Ioffe−Regel criterion, while absorption has to be negligible [15] , [16] , [17] , [18] . On the contrary, two-dimensional (2D), or transverse, localization [19] is always obtained in sufficiently large samples and has various analogies with the focusing through adaptive processes: they are both coherent phenomena and allow to trap light in a tiny spot. Transverse localization [19] occurs in systems disordered in the plane perpendicular to the direction of propagation: it has been demonstrated in arrays [20] , in optical lattices [21] , and in plastic [22] and glass [23] fibres, while the role of transverse localization (TL) in speckle focusing has never been previously investigated. Here we study the interplay between the focusing process and Anderson localization and demonstrate that the absence of diffusion cooperates with the optimization protocol to improve focusing effectiveness. Transverse Anderson localization in optical fibres We use an optical fibre (without cladding) with transverse disorder and binary refractive index modulation [9] , [22] , [24] which supports transversal Anderson localization (see inset of Fig. 1 and Methods section). 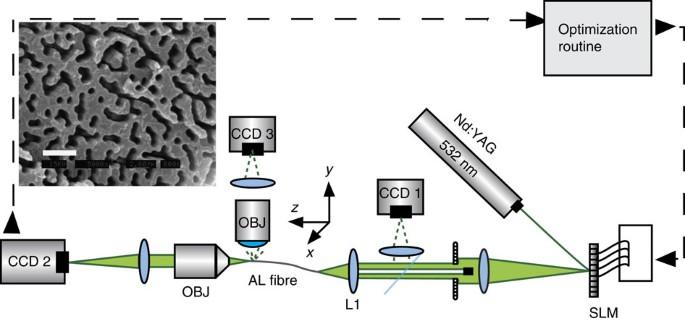Figure 1: Experimental apparatus. Light from a solid state ND:YAG laser is reflected by an SLM in phase-only configuration obtained by blocking the first diffracted order by a beam stop. Modulated light is coupled by the lens L1 onto the fibre. Input and output faces of the fibre are imaged by microscopy objectives (OBJ) on CCD 1 and CCD 2, respectively. A computer-aided feedback controls the SLM. The lateral side of the fibre tip is imaged on CCD 3. The inset shows a scanning electron microscope image of the fibre tip, in which darker regions correspond to PMMA. White scale bar, 4 μm. Figure 1: Experimental apparatus. Light from a solid state ND:YAG laser is reflected by an SLM in phase-only configuration obtained by blocking the first diffracted order by a beam stop. Modulated light is coupled by the lens L1 onto the fibre. Input and output faces of the fibre are imaged by microscopy objectives (OBJ) on CCD 1 and CCD 2, respectively. A computer-aided feedback controls the SLM. The lateral side of the fibre tip is imaged on CCD 3. The inset shows a scanning electron microscope image of the fibre tip, in which darker regions correspond to PMMA. White scale bar, 4 μm. Full size image Independently of the spatial shape of the input beam, some particular hotspots at fixed positions in the fibre output are observed, as in Fig. 2a,b , which show the transmitted intensity from the output face of the fibre. 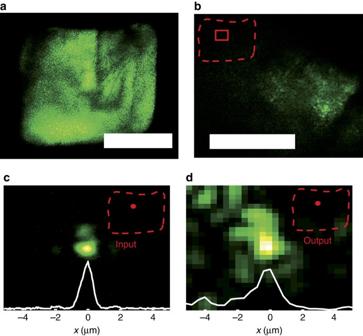Figure 2: Light transmission in the disordered fibres. (a) Laser at the fibre output (side 250 μm); scale, 130 μm. (b) As ina, averaged over 500 random input and zoomed on the position indicated in the red sketches; scale, 27 μm. (c) Laser at the fibre input face in the single-mode injection (0.7 μm input spot); (d) output of the fibre corresponding to the input condition inc. The location of the hotspots in the fibre is sketched in the insets. Figure 2b is obtained by averaging 500 random input configurations realized by a random SLM phase mask producing a 60-μm speckled spot at the fibre entrance (see also Fig. 3a,b ). The presence of hotspots appearing at fixed positions independently of the input mask is connected with extremely efficient transport channels [4] . The high-transmitting channels are Anderson modes of the fibres, that is, TLs that retain a fixed transverse profile along propagation. This is demonstrated by injecting light by a long working-distance objective (numerical aperture 0.8, resulting focused spot size 0.7 μm), which feeds selectively a single mode. In this configuration the input and the output spots are similar in size ( Fig. 2c,d ), and appear at the same transverse location in the fibre. This confirms that the excited mode is an eigenmode of the fibre, and its shape and position are not affected by the propagation. Figure 2: Light transmission in the disordered fibres. ( a ) Laser at the fibre output (side 250 μm); scale, 130 μm. ( b ) As in a , averaged over 500 random input and zoomed on the position indicated in the red sketches; scale, 27 μm. ( c ) Laser at the fibre input face in the single-mode injection (0.7 μm input spot); ( d ) output of the fibre corresponding to the input condition in c . The location of the hotspots in the fibre is sketched in the insets. 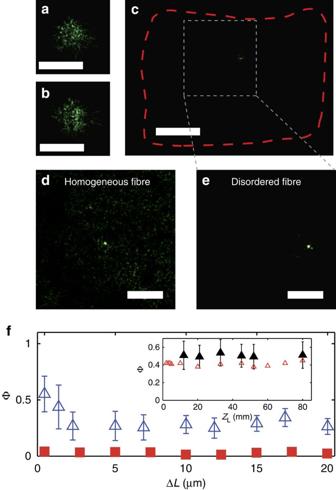Figure 3: Adaptive focusing in the Anderson regime. Input spot on the fibre before (a) and after (b) the optimization procedure by CCD 1 (scale, 60 μm). (c) Fibre output after the optimization procedure by CCD 2 (scale, 66 μm). (d) Fibre output with magnification higher thancfor a PMMA-homogeneous fibre; (e) as indfor an ALF (scale, 28 μm (e,d)). (f) Focus efficiency Φ as a function of the distance ΔLfrom an output hotspot for the homogeneous PMMA fibre (full squares) and for the ALF (open circles). Error bars are given by the statistics on five samples, and are smaller than symbols in the homogeneous fibre. The inset shows Φ as a function of the fibre lengthZL, measured experimentally (full triangles) and numerically calculated (open triangles,V0=100). Full size image Figure 3: Adaptive focusing in the Anderson regime. Input spot on the fibre before ( a ) and after ( b ) the optimization procedure by CCD 1 (scale, 60 μm). ( c ) Fibre output after the optimization procedure by CCD 2 (scale, 66 μm). ( d ) Fibre output with magnification higher than c for a PMMA-homogeneous fibre; ( e ) as in d for an ALF (scale, 28 μm ( e , d )). ( f ) Focus efficiency Φ as a function of the distance Δ L from an output hotspot for the homogeneous PMMA fibre (full squares) and for the ALF (open circles). Error bars are given by the statistics on five samples, and are smaller than symbols in the homogeneous fibre. The inset shows Φ as a function of the fibre length Z L , measured experimentally (full triangles) and numerically calculated (open triangles, V 0 =100). Full size image Light focusing in the Anderson regime Having located such efficient channels, we applied a feedback algorithm to improve the intensity in one of the observed hotspots. Our approach is a standard one, very similar to that described in ref. 25 : a random phase shift is applied to a segment of the SLM, which is divided into a 23 × 23 matrix composed by 529 segments. The CCD 1 in Fig. 1 grabs an image of the output and the algorithm retains the change in the phase mask only if the intensity in the hotspot increases, otherwise the previous phase shift is restored. At the end of the optimization procedure (after 529 steps) more than one half of the fibre output has been channelled into the target point, that is, into a 4-μm area (fibre lateral side W =250 μm). The input speckled beam (60 μm waist, obtained by a 50-mm focal lens), is shown in Fig. 3a (before the optimization) and Fig. 3b (at the end of the optimization). Figure 3c shows the image of the output-focused beam, and demonstrates that, in the Anderson regime, one half of the transmitted energy is focused in a 2-μm 2 squared area centred at the target, the ratio of the intensity at focus with respect to the average background is 10 4 . For comparison, we repeated the experiment by using a homogeneous disorder-free standard fibre and found very different results: the optimized focused spot contains only 1% of the total transmitted intensity, and the ratio of the intensity at focus with respect to the average background is of the order of 50; this is a result comparable to the state of the art in multimode fibres [26] , [27] , [28] . The same comparison cannot be done with photonic crystal fibres, which typically support few modes, thus making impossible the optimization protocol. The approach proposed here has several advantages also when compared with fibre bundles: the absence of an alignment requiring mechanical movement of the optics and a larger set of possible outputs. All the possible positions of the output facet may be targeted also simultaneously generating multiple foci. Images of the focus for the homogeneous polymethyl methacrylate (PMMA) fibre and for the Anderson fibre (ALF) are shown in Fig. 3d,e , respectively. A further comparison between various cases is in Fig. 4 , in which the profiles of the focus in various configurations are reported. At variance with the standard PMMA fibre, the presence of TL introduces a strong dishomogeneity of the response in the transverse direction. We performed a set of measurements (shown in Fig. 3f ) with variable distance Δ L from a high-transmitting transport channel, determined by the position of the output hotspots as described above. Specifically, instead of maximizing the intensity in correspondence of a chosen hotspot, we maximized the intensity at a distance Δ L from it and measured the focusing efficiency, defined as the ratio Φ between the power channelled in this shifted position (at the end of the optimization procedure) and the total output power from the fibre. The result in Fig. 3f shows that Φ rapidly decreases when moving far away from the hotspot, which hence represents the most efficient position of the focusing (and corresponds to a TL). On the contrary, the homogeneous fibre (red squares in Fig. 3f ) shows no significant variation of Φ in terms of Δ L . 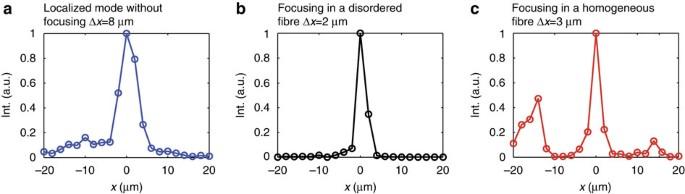Figure 4: Intensity profile of the focus. Profile of a localized mode (a) without optimization and (b) after the optimization procedure. (c) A focused mode in a homogeneous fibre; note the background. Figure 4: Intensity profile of the focus. Profile of a localized mode ( a ) without optimization and ( b ) after the optimization procedure. ( c ) A focused mode in a homogeneous fibre; note the background. Full size image This difference is ascribed to the presence of TL. To demonstrate that the propagation-invariant TL is the leading mechanism to concentrate light at the target point, we repeated the focusing experiments with fibres with varying length Z L . The inset in Fig. 3f shows that Φ is nearly independent of Z L , as is also confirmed by the results from the numerical simulation described below. The most effective focusing in the disordered case is due to the presence of the Anderson localization that inhibits light diffusion and practically eliminates the background speckle pattern. We stress that the TL focusing action is concomitant with the standard focusing action, which involves all the modes of the fibres and results in an enhancement of the intensity at the focus. Numerical simulation of adaptive focusing To further confirm this scenario, we resorted to the numerical simulation of the paraxial equation approximating the propagation of an optical field A (with I=|A| 2 the beam intensity) in the ALF [29] . In dimensionless units this equation reads as with V =−2 k 2 W 2 Δ n / n 0 , a =A/√I 0 , I 0 being a reference intensity, k =2 πn 0 / λ and n 0 the average refractive index. The transverse disorder is given by a term representing the random fluctuations of the refractive index in the transverse plane Δ n =Δ n ( X , Y ), and z = Z /(2 kW 2 ) and ( x , y )=( X / W , Y / W ). Equation (1) is an approximate scalar model for beam propagation in a high index contrast ALF. However, while fully vectorial calculations allow determining the supported mode profiles, the simulation of the optimization procedure and beam propagation is computationally prohibitive beyond the scalar approximation in equation (1). The transverse bound states (2D Anderson localizations) in this simplified model are given by a = ϕ n ( x , y )exp( iE n z ) with Because of the mentioned computational limitations, we approximate the disorder distribution by Gaussian random potential, such that . We remark that the distribution of the disorder is coarse-grained in the numerical simulations by the adopted discretization and by retaining as independent Gaussian variables the noise values in different grid points. We verified that the discretization does not affect the reported results by increasing the number of grid points in the numerical simulations. We also considered binary random potentials (not reported) with results similar to what follows. The Gaussian potential is also included in a rectangular well to account for the interface between the fibre and air. The strength of the potential V 0 is determined by the refractive index contrast: the index jump between polystyrene (PS) and PMMA is Δ n =0.1 as the latter varies on a spatial scale Δ D =1 μm of the order of λ , we have V 0 =2 k 2 W 2 Δ D Δ n / n 0 , which gives V 0 ≅ 100 for our fibre; for comparison we take V 0 =10 for the weak disorder cases. In our trials, we varied V 0 in a range of two decades and found no qualitative changes with respect to the representative cases reported in the following; we stress that the considered propagation distances correspond to those in our experiments (in our normalized units z =1 corresponds to Z L ≅ 1 m). We first determine the 2D eigenmodes in our simplified model from equation (2), as given in Fig. 5a ( Fig. 5d ) for the low (high)-index contrast case. The mode with the stronger localization (ground state) is chosen as the target for the optimization. By solving equation (1), the field profile at each point ( x , y and z ) is calculated; the input condition is generated as done in the experiments and results in speckled beam are shown in Fig. 5b ( Fig. 5e ) for the low (high)-index contrast. After a random modification of the phase at the input, the solution of equation (1) is calculated, and the change is retained if the intensity at the target point increases. The output profiles are given in Fig. 5c,f . 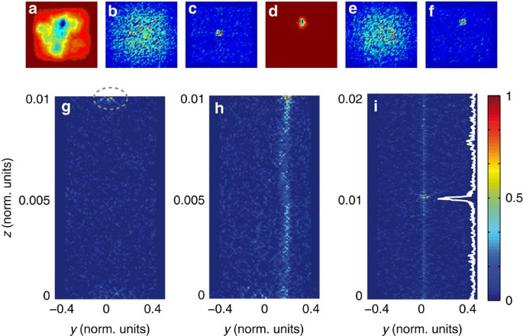Figure 5: Numerical simulations. In the low index contrast (V0=10) configuration: (a) ground state; (b) input after optimization; (c) output after optimization. (g) Intensity distribution in the section of fibre in correspondence of the output spot along propagation direction; note that the focusing occurs in the last part of propagation as indicated by the dashed circle. Results after equation (1) for high index contrast (V0=100): (d) ground state; (e) input after optimization; (f) output after optimization. (h) Intensity distribution in the section of fibre in correspondence of the output spot along propagation direction. Note that the localization since the beginning of propagation and further enhanced at the end. (i) As inhfor a doubled propagation length and with the optimization target located in the middle of the fibre. The white line is the intensity profile in correspondence of the focus versusz. Figure 5: Numerical simulations. In the low index contrast ( V 0 =10) configuration: ( a ) ground state; ( b ) input after optimization; ( c ) output after optimization. ( g ) Intensity distribution in the section of fibre in correspondence of the output spot along propagation direction; note that the focusing occurs in the last part of propagation as indicated by the dashed circle. Results after equation (1) for high index contrast ( V 0 =100): ( d ) ground state; ( e ) input after optimization; ( f ) output after optimization. ( h ) Intensity distribution in the section of fibre in correspondence of the output spot along propagation direction. Note that the localization since the beginning of propagation and further enhanced at the end. ( i ) As in h for a doubled propagation length and with the optimization target located in the middle of the fibre. The white line is the intensity profile in correspondence of the focus versus z . Full size image When the index contrast is very small (that is, far from the strong localization condition), the focusing appears only at the very end of the fibre ( Fig. 5g ), that is at a well-defined z , as it occurs in 3D with standard materials [1] , or in multimode optical fibres [26] . When the degree of localization is strong ( Fig. 5h ), the focus appears in correspondence of a TL, propagating along the direction z , being enhanced at the fibre tip. In Fig. 5i we show the intensity profile after an optimization for a target located in the middle of fibre, and found a pronounced intensity peak in the focus. This shows that most of the energy is carried by the TL located at the target, and that the other modes interfere constructively to enhance the local optimized intensity. As in experiments, the numerical simulations furnish an efficiency Φ independent of the fibre length (see inset of Fig. 3f ). The numerically calculated Φ is found to be slightly smaller than the experimentally measured value owing to the limited resolution of the simulations, where we also considered very small fibre lengths not accessible in the experiments ( Z L <12 mm in Fig. 3f ). We experimentally verified the existence of such propagating mode appearing together with the focus in the ALF by measuring the light scattered at one side of the fibre, by using a microscope and CCD 3 (see Fig. 1 ). Results are reported in Fig. 6 , where the arrow indicates the direction of light propagation. 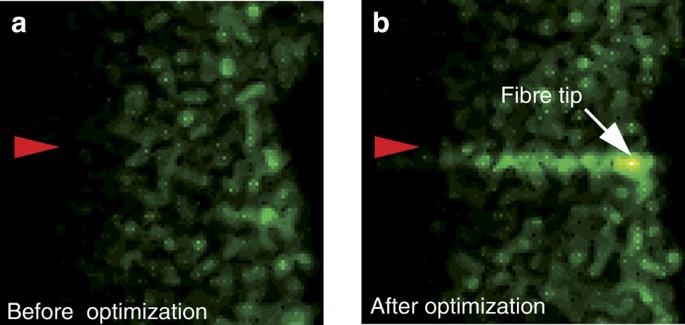Figure 6: Localized mode and adaptive focus. Light scattered from the side of the fibre in correspondence of the exit tip (a) before the optimization process and (b) after the optimization process. The side of the panels is 160 μm. Figure 6a shows the image of the ALF side before the focusing-optimization process and Fig. 6b shows the same fibre section at the end of the focusing-optimization process. In the latter case, intensity is increased not only at the fibre end-tip but also along the z axis. Figure 6: Localized mode and adaptive focus. Light scattered from the side of the fibre in correspondence of the exit tip ( a ) before the optimization process and ( b ) after the optimization process. The side of the panels is 160 μm. Full size image We investigated light focusing in random media by an adaptive technique in the presence of transverse Anderson localization. By applying an iterative optimization process we were able to feed a localized mode by a spatially modulated beam. The quality of the obtained focus differs strongly from what is reported in 3D disordered structures and in standard fibres, because light couples to localized modes travelling for centimetres. We found that the inhibition of diffusion imposed by the Anderson regime boosts the amount of light coupled to the target, lowering the detrimental contribution to the focusing due to the background speckle pattern by several orders of magnitude. The transversal localization hence non-trivially cooperates in the focusing action, and two mechanisms are found to occur: on one hand, the TL located at the target point transports most of the energy; on the other hand, the other modes interfere locally and enhance the intensity. At variance with other imaging fibre technologies (like fibre endoscopes or fibre bundles), modes of an ALF are coupled allowing adaptive focusing to produce a focused spot (with 2 μm size) at any user-defined position (which is not possible in systems with uncoupled modes). With respect to multimode fibres, the ALF enables to gather a larger fraction of the transmitted light at the target position with lower background intensity. The resulting focusing efficiency is found to be nearly independent of the fibre length, and this may ultimately lead to a variety of applications based on the transport and focusing of light at specific points also located in distant positions within the disordered matter. Disordered optical fibres We use an optical fibre (without cladding) with transverse disorder and binary refractive index modulation [9] , [22] , [24] (see inset of Fig. 1 ). The index contrast of the order of 0.1 results from the difference between PS (refractive index n =1.59) and PMMA ( n =1.49). We estimate the value of losses in 0.5 Db cm −1 . This value will be further decreased of at least two orders of magnitude exploiting advanced fabrication techniques. Moreover, a relevant part of the losses is due to the input and output coupling and can be reduced by improving the fibre-cutting procedure. The disordered fibre has been fabricated by melding 40,000 strands of PS and 40,000 strands of PMMA. The mixture of strands was fused together and redrawn to a square-shaped fibre with a lateral size W =250 μm (ref. 22 ). Samples have length Z L between 1.2 and 8 cm. Light generated by a continuous wave laser with wavelength λ =532 nm (vertical polarization) is injected in the system after being modulated by an SLM in the phase-only configuration (experimental set-up is shown in Fig. 1 ). Figure 2a shows the fibre output when the input is completely illuminated (horizontal polarization is retrieved to eliminate ballistic light). The focusing effect is found to be independent of the input polarization. Such a structure supports strong localization (as already demonstrated in ref. 22 ), having a refractive index mismatch three orders of magnitude larger than in the seminal experiment of ref. 21 , and also allows image transmission [30] . How to cite this article: Leonetti, M. et al. Light focusing in the Anderson regime. Nat. Commun. 5:4534 doi: 10.1038/ncomms5534 (2014).